Radial symmetry in a chimeric glutamate receptor pore Ionotropic glutamate receptors comprise two conformationally different A/C and B/D subunit pairs. Closed channels exhibit fourfold radial symmetry in the transmembrane domain (TMD) but transition to twofold dimer-of-dimers symmetry for extracellular ligand binding and N-terminal domains. Here, to evaluate symmetry in open pores we analysed interaction between the Q/R editing site near the pore loop apex and the transmembrane M3 helix of kainate receptor subunit GluK2. Chimeric subunits that combined the GluK2 TMD with extracellular segments from NMDA receptors, which are obligate heteromers, yielded channels made up of A/C and B/D subunit pairs with distinct substitutions along M3 and/or Q/R site editing status, in an otherwise identical homotetrameric TMD. Our results indicate that Q/R site interaction with M3 occurs within individual subunits and is essentially the same for both A/C and B/D subunit conformations, suggesting that fourfold pore symmetry persists in the open state. Ionotropic glutamate receptors (iGluRs) are ligand-gated ion channels that mediate excitatory synaptic transmission throughout the central nervous system. Aberrant activation of these receptors is implicated in a number of pathological situations, which has motivated intense effort to understand their operation and to devise therapeutic interventions that might allow for the regulation of iGluR activity [1] . The three main iGluR subtypes, named for the agonists N -methyl- D -aspartate (NMDA), α-amino-3-hydroxy-5-methyl-4-isoxazolepropionic acid (AMPA) and kainate (KA), are made up of distinct sets of homologous subunits that combine as homo or heteromeric tetramers to form an ion conducting pathway through the membrane [1] . X-ray crystallography of subunit subdomains [2] and of an intact homomeric AMPA receptor in the closed state [3] has revealed a modular structure with twofold symmetry in the extracellular amino terminal and ligand-binding domains (ATD and LBD) and apparent fourfold symmetry in the channel-forming transmembrane domain (TMD) ( Fig. 1 ). The iGluR channels exhibit a pore-helix and selectivity filter flanked by two transmembrane helices as originally described for the KcsA channel [4] , but with inverted topology. In addition, all eukaryotic iGluR subunits include an additional transmembrane helix (M4) that is essential for channel function [5] , [6] , [7] . In contrast to potassium channels and most other members of this ion channel superfamily, the pore loop in iGluRs is on the cytoplasmic face of the channel and the inner helix bundle crossing, believed to form the gate to ion passage, faces the extracellular side and connects to the LBD via short linkers. Motion of the LBD coincident with agonist binding is thought to pull on the linkers, inducing a conformational change in the TMD that opens the channel. Once open, iGluRs conduct monovalent cations and in some cases calcium ions [1] . 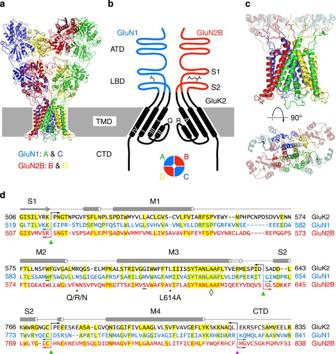Figure 1: Glutamate receptor domain structure. (a) Chimeric glutamate receptor homology model based on the homomeric GluA2 AMPA receptor closed state X-ray structure (Sobolevskyet al.3) illustrating the amino-terminal domain (ATD), ligand-binding domain (LBD) and transmembrane domain (TMD). The cytoplasmic carboxy terminal domain (CTD) was not resolved or modelled. Each subunit is shown in a different colour. In wild-type NMDA receptors GluN1 and GluN2B subunits are in the A/C and B/D conformations, respectively. (b) Diagram of the four domains in two chimeric subunits of a heteromeric receptor highlighting the pore loop and M1-M4 alpha helices in the TMD derived from KA receptor subunit GluK2 (white roman numerals I, II, III, IV). Left hand subunit is unedited (Q) at the apex of the pore loop and wild type L614 in M3 at the level of the central cavity. Right hand subunit is edited (R) and mutated (L614A) in M3. Subunits with N1 and N2B extracellular domains are presumed to be adjacent in functional tetramers (below), but for clarity are positioned opposite each other in the diagram. (c) Enlarged side and axial views of the homology model showing the lower portion of the LBD in faint teal (GluN1) and red (GluN2B), as well as the TMD and linkers from GluK2 in full colour. The view down the central axis from the extracellular domains illustrates differences in the A/C and B/D linkers. (d) Sequence alignment for chimeric GluN1 and GluN2B with GluK2. Green triangles indicate the position of joints in the chimeric subunits. The purple triangle indicates an additional joint for subunits that only included the TMD from GluK2. Numbering is for the mature wild-type proteins. Secondary structure is shown as cylinders (α-helices), arrows (β-strands) and lines (loops) in grey above the sequence. * indicates the Q/R/N site in the pore loop and the GluK2 L614A mutation site in M3.◊indicates the M3 Ala at the middle of the bundle crossing. The W in M2 of GluN1 and the S in M3 of GluN2B that interact with each other (Siegler Retchlesset al.14) are underlined. Figure 1: Glutamate receptor domain structure. ( a ) Chimeric glutamate receptor homology model based on the homomeric GluA2 AMPA receptor closed state X-ray structure (Sobolevsky et al. [3] ) illustrating the amino-terminal domain (ATD), ligand-binding domain (LBD) and transmembrane domain (TMD). The cytoplasmic carboxy terminal domain (CTD) was not resolved or modelled. Each subunit is shown in a different colour. In wild-type NMDA receptors GluN1 and GluN2B subunits are in the A/C and B/D conformations, respectively. ( b ) Diagram of the four domains in two chimeric subunits of a heteromeric receptor highlighting the pore loop and M1-M4 alpha helices in the TMD derived from KA receptor subunit GluK2 (white roman numerals I, II, III, IV). Left hand subunit is unedited (Q) at the apex of the pore loop and wild type L614 in M3 at the level of the central cavity. Right hand subunit is edited (R) and mutated (L614A) in M3. Subunits with N1 and N2B extracellular domains are presumed to be adjacent in functional tetramers ( below ), but for clarity are positioned opposite each other in the diagram. ( c ) Enlarged side and axial views of the homology model showing the lower portion of the LBD in faint teal (GluN1) and red (GluN2B), as well as the TMD and linkers from GluK2 in full colour. The view down the central axis from the extracellular domains illustrates differences in the A/C and B/D linkers. ( d ) Sequence alignment for chimeric GluN1 and GluN2B with GluK2. Green triangles indicate the position of joints in the chimeric subunits. The purple triangle indicates an additional joint for subunits that only included the TMD from GluK2. Numbering is for the mature wild-type proteins. Secondary structure is shown as cylinders (α-helices), arrows (β-strands) and lines (loops) in grey above the sequence. * indicates the Q/R/N site in the pore loop and the GluK2 L614A mutation site in M3. ◊ indicates the M3 Ala at the middle of the bundle crossing. The W in M2 of GluN1 and the S in M3 of GluN2B that interact with each other (Siegler Retchless et al. [14] ) are underlined. Full size image A striking feature of the intact homomeric GluA2 crystal structure [3] is the presence of two distinct subunit configurations, with identical A/C and B/D subunit pairs arranged diagonally across from each other within the TMD. In the closed state structure, the transition from twofold to fourfold symmetry occurs within a narrow zone near the extracellular membrane surface where the linkers connect the LBD and TMD [3] . It remains unclear, however, whether this abrupt symmetry transition persists when channels open or desensitize. Indeed, several lines of evidence suggest that in the open state there may be asymmetries between the A/C and B/D subunit pairs, at least near the bundle crossing where the extracellular ends of the inner (M3) helix make close contact to occlude ion passage. For example, studies of heteromeric NMDA receptors with inner helix cysteine substitutions in and around the highly conserved SYTANLAAF motif have demonstrated asymmetric modification for homologous positions of GluN1 versus GluN2 subunits [8] , suggesting an offset of the A/C (GluN1) relative to B/D (GluN2) subunit pairs. In addition, homomeric GluA1 AMPA receptors with cysteine substitutions in this segment exhibit block by cadmium ions that is consistent with twofold symmetry in the open state [9] . More recent experiments on both AMPA [10] and NMDA [11] receptors have provided evidence for differences between the A/C and B/D subunit pairs in the extent and timing of gating-associated movements. It remains to be determined whether these apparent asymmetries are confined to the extracellular portions of M3, close to the linkers connecting to the LBD, or whether the entire TMD converts to twofold symmetry when channels open and/or desensitize [12] . To begin addressing this question, we have analysed an interaction that was recently discovered between residues along the inner (M3) helix and the Q/R site near the apex of the pore loop of homomeric GluK2 KA receptors [13] . The Q/R site is a location where RNA editing can alter the primary amino-acid sequence, replacing a polar, but uncharged glutamine (Q) encoded by genomic DNA with a positively charged arginine (R). Such editing occurs in the KA receptor GluK1 and GluK2 subunits, as well as the GluA2 subunit of AMPA receptors. The homologous position remains a Q in all other AMPA and KA receptor subunits and an asparagine in all GluN1 and GluN2 NMDA receptor subunits [1] . Q/R site editing controls a variety of channel properties [1] including ion selectivity and unitary conductance, as well as susceptibility to inhibition by polyamines and by cis -unsaturated fatty acids such as arachidonic and docosahexaenoic acid (AA and DHA). As shown by recent work [13] , the GluK2 pore loop Q/R site interacts with several residues along the inner (M3) helix, most notably with the side chain at position L614 at the level of the central cavity ( Fig. 1 ). Moreover, exposure to DHA enhances the strength of this energetic coupling. For example, in control conditions Q/R site editing interacts with L614V or D substitutions with a coupling energy of ~2.5 k T, and treatment with DHA increases the coupling in both cases by an additional 3 k T. The GluK2(R) L614A substitution mutant displays the largest change with DHA treatment. Whereas wild-type homomeric edited GluK2(R) channels are more than 80% inhibited by exposure to DHA, when editing is combined with the L614A substitution DHA treatment potentiates agonist-evoked currents by ~10-fold. Although these results in homomeric channels demonstrated strong interaction between the Q/R site and M3 helix, they did not reveal whether the interaction is equivalent for all four subunits or whether there are substantial differences between the relative contributions of the A/C and B/D subunit pairs. In addition, work to date has not determined whether the Q/R site to M3 interaction occurs within an individual subunit or across the boundary between two adjacent subunits [13] , [14] . In this study, to address these questions we have constructed chimeric channels that combine the TMD and cytoplasmic carboxy terminal domain (CTD) of the GluK2 kainate receptor subunit with the extracellular ATD and LBD of NMDA receptor subunits GluN1 and GluN2B. Because NMDA receptors are obligate heteromers [1] and the extracellular domains are strongly implicated in specifying the heteromeric arrangement of subunits within tetrameric channels [15] , we reasoned that functional channels would only be generated when both GluN1/GluK2 and GluN2B/GluK2 chimera were co-expressed, which turned out to be the case. In this way we were able to construct channels with A/C and B/D subunits that differed in their Q/R editing or M3 substitutions, or both. Using this approach, we show that interactions between the Q/R site and M3 helix occur within each subunit, not between adjacent subunits, and that pore loop to M3 interactions within the A/C and B/D subunit pairs make nearly equal contributions to the potentiation elicited by treatment with DHA, suggesting that the fourfold radial symmetry observed for the closed state TMD is preserved when channels open, at least up to the level of the central cavity. Chimeric subunits with a kainate receptor pore Previous efforts to transplant just the M1 to M3 segment between NMDA and KA receptor subunits met with limited success [16] , probably because interaction of the M1 to M3 pore with the M4 transmembrane helix is now recognized to be essential for channel assembly [7] and/or function [5] , [6] . Therefore, we combined the entire KA receptor TMD including the linkers to the LBD, as well as the CTD, with the extracellular domains from NMDA receptor subunits GluN1 and GluN2B ( Fig. 1 ). In wild-type NMDA receptors glutamate or NMDA binds to the GluN2 subunit, whereas the co-agonist glycine or D -serine binds to GluN1 (ref. 1 ). In addition, recent work [17] , [18] supports the assignment [3] of GluN1 to the A/C configuration and GluN2 to the B/D configuration (but see ref. 19 ). As shown in Fig. 2a expression of each chimeric subunit alone, in either the unedited (Q) or edited (R) form, failed to generate functional homomeric channels; however, co-expression of the GluN1-GluK2 pore (N1/K2) and GluN2B-GluK2 pore (N2B/K2) chimeric subunits together resulted in channels that were activated by application of NMDA and the co-agonist glycine [20] , [21] . As for wild-type full-length GluK2, when both subunits were unedited (Q) in the pore loop, the resulting channels displayed bi-rectifying current-voltage relations ( Fig. 2b ) indicative of voltage-dependent block by cytoplasmic polyamines [1] . In contrast, if one or both subunits was in the edited (R) form, then polyamine block was diminished and the IV relation was linear ( Fig. 2c–e ), or showed slight outward rectification [22] . Importantly, exposure to DHA strongly inhibited channels in which all of the subunits were edited (R) in the pore loop but caused little or no change in channels with either or both subunits in the unedited (Q) form ( P <0.0001, one-way ANOVA with post hoc Student-Newman-Keuls comparison) ( Fig. 3 ), which is identical to the pattern of DHA modulation observed for wild-type full-length recombinant heteromeric kainate receptors [23] ( Fig. 3c ). A similar outcome was obtained with constructs in which the CTD, as well as the ATD and LBD, came from GluN1 and GluN2B. 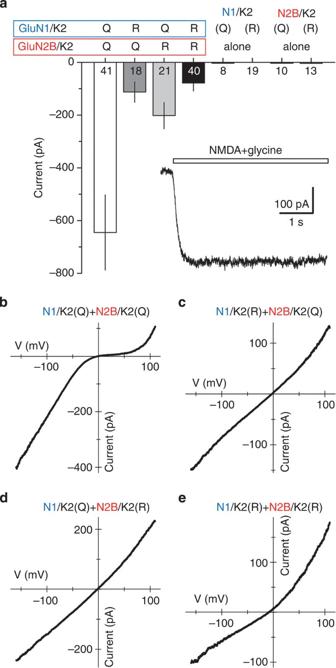Figure 2: Whole-cell current and current-voltage relations for channels with kainate receptor pores. (a) Whole-cell current (mean±s.e.m.) evoked by 10 μM NMDA plus 10 μM glycine in HEK 293 cells transfected with edited (R) or unedited (Q) N1/K2 and N2B/K2 chimeric subunits. Agonist application did not elicit current in cells transfected with the N1/K2(Q/R) or N2B/K2(Q/R) subunits alone. Sample size is shown for each bar. (inset) Current recorded from a cell transfected with N1/K2(Q)+N2B/K2(Q). (b–e) Whole-cell currents evoked by 10 μM NMDA and 10 μM glycine as the membrane potential was ramped from −160 to +110 mV at 0.75 mv ms−1. (b) Birectification of current mediated by N1/K2(Q)+N2B/K2(Q) reflects block by endogenous polyamines, as well as 20 μM spermine added to the internal solution, with relief of block as the polyamines permeate the channel at positive potentials. Polyamine block was eliminated by Arg substitution at the Q/R site of either the N1/K2 (c) or N2B/K2 (d) subunit, or both subunits (e). Figure 2: Whole-cell current and current-voltage relations for channels with kainate receptor pores. ( a ) Whole-cell current (mean±s.e.m.) evoked by 10 μM NMDA plus 10 μM glycine in HEK 293 cells transfected with edited (R) or unedited (Q) N1/K2 and N2B/K2 chimeric subunits. Agonist application did not elicit current in cells transfected with the N1/K2(Q/R) or N2B/K2(Q/R) subunits alone. Sample size is shown for each bar. ( inset ) Current recorded from a cell transfected with N1/K2(Q)+N2B/K2(Q). ( b – e ) Whole-cell currents evoked by 10 μM NMDA and 10 μM glycine as the membrane potential was ramped from −160 to +110 mV at 0.75 mv ms −1 . ( b ) Birectification of current mediated by N1/K2(Q)+N2B/K2(Q) reflects block by endogenous polyamines, as well as 20 μM spermine added to the internal solution, with relief of block as the polyamines permeate the channel at positive potentials. Polyamine block was eliminated by Arg substitution at the Q/R site of either the N1/K2 ( c ) or N2B/K2 ( d ) subunit, or both subunits ( e ). 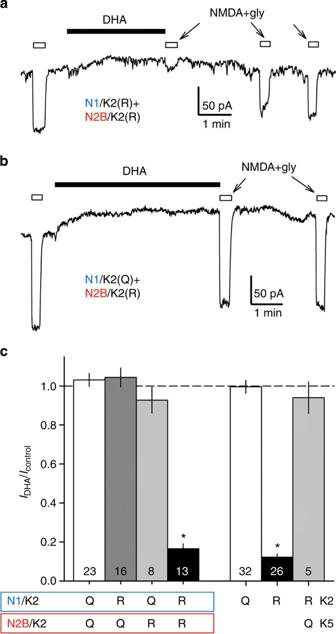Figure 3: Selective DHA inhibition of fully edited chimeric receptors. Whole-cell current evoked by 10 μM NMDA and 10 μM glycine (open bars) at −80 mV before and after exposure to 30 μM DHA (solid bar) in a cell transfected with fully edited N1/K2(R)+N2B/K2(R) subunits (a) and in a cell that received N1/K2(Q)+N2B/K2(R) (b). (c) Plot of current evoked immediately after exposure to DHA as a fraction of control current before DHA (mean±s.e.m.) for the four chimeric combinations and, for comparison, wild-type homomeric GluK2(Q) and (R) and heteromeric GluK2(R)+GluK5(Q). Sample size is shown for each bar. * significantly different from N1/K2(Q)+N2B/K2(Q) and homomeric GluK2(Q) (P<0.0001, one-way ANOVA withpost hocStudent-Newman-Keuls comparison). Full size image Figure 3: Selective DHA inhibition of fully edited chimeric receptors. Whole-cell current evoked by 10 μM NMDA and 10 μM glycine (open bars) at −80 mV before and after exposure to 30 μM DHA (solid bar) in a cell transfected with fully edited N1/K2(R)+N2B/K2(R) subunits ( a ) and in a cell that received N1/K2(Q)+N2B/K2(R) ( b ). ( c ) Plot of current evoked immediately after exposure to DHA as a fraction of control current before DHA (mean±s.e.m.) for the four chimeric combinations and, for comparison, wild-type homomeric GluK2(Q) and (R) and heteromeric GluK2(R)+GluK5(Q). Sample size is shown for each bar. * significantly different from N1/K2(Q)+N2B/K2(Q) and homomeric GluK2(Q) ( P <0.0001, one-way ANOVA with post hoc Student-Newman-Keuls comparison). Full size image Taken together, these results demonstrate that the kainate receptor TMD is sufficient to determine the effect of DHA exposure: inhibition when all four subunits are edited (R), but neither inhibition nor potentiation when one or both subunits is unedited (Q). Thus, the NMDA receptor ATD and LBD domains effectively activate all of the edited and unedited GluK2 pore combinations but are not able to prevent inhibition of R/R pores by DHA or to induce potentiation of Q/R, R/Q or Q/Q pores [24] , [25] . Collectively, these results strongly suggest that AA and DHA act by partitioning into the membrane and directly or indirectly modifying conformational changes in the TMD associated with channel opening. Q/R site interaction with the M3 helix Recent work on homomeric GluK2 KA receptors has demonstrated that several amino acids along the inner transmembrane helix (M3) interact selectively with the Arg side chain at the Q/R site in fully edited channels [13] . In particular, a number of substitutions at position L614 completely reverse the effect of DHA exposure on GluK2(R), while having little or no effect on GluK2(Q). Substitution of L614 with alanine had the largest effect, converting ~90% inhibition of wild-type GluK2(R) to approximately 10-fold potentiation for homomeric GluK2(R)L614A (ref. 13 ). To determine the relative contribution of the A/C and B/D subunit pairs to this interaction and to test whether it occurs between adjacent subunits or within individual subunits, we made Q and R forms of both GluN1/K2 and GluN2B/K2 each bearing alanine substituted for the leucine homologous to L614 in full-length GluK2 (henceforth referred to as L614A substitutions in the chimeric subunits). As shown in Fig. 4 , all 12 of the possible heteromeric combinations of mutant and non-mutant subunits were functional and a clear pattern emerged for modulation of channel function by DHA: first, the strongest potentiation by DHA (>10-fold) occurred when all four subunits were both edited (R) and mutated (L614A); second, intermediate potentiation (two- to fourfold) was observed when one of the two chimeric subunits was both edited (R) and mutated (L614A); third, less than 1.5-fold potentiation occurred when the L614A mutation was only present in unedited (Q) subunits ( P <0.0001, one-way ANOVA with post hoc Student-Newman-Keuls comparison). 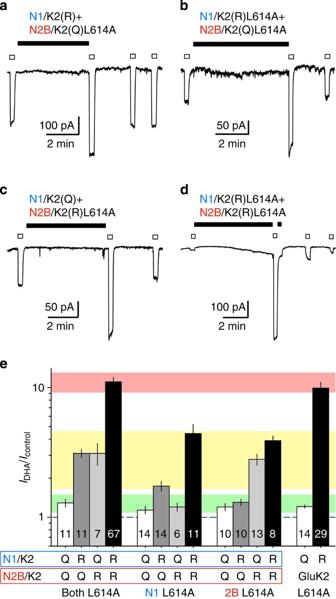Figure 4: Intrasubunit interaction between the pore loop and M3 helix. Whole-cell current evoked by 10 μM NMDA and 10 μM glycine (open bars) at −80 mV before and after exposure to 30 μM DHA (solid bar) in cells co-transfected with N1/K2(R)+N2B/K2(Q)L614A (a), N1/K2(R)L614A+N2B/K2(Q)L614A (b), N1/K2(Q)+N2B/K2(R)L614A (c), or N1/K2(R)L614A+N2B/K2(R)L614A (d). (e) Plot of current evoked immediately after exposure to DHA as a fraction of control current before DHA (mean±s.e.m.) for the 12 chimeric constructs and, for comparison, homomeric L614A mutants of GluK2(Q) and (R). Sample size is shown for each bar. Note the logarithmic scale. DHA had minimal effect when L614A and Q to R editing were not present on the same chimeric subunit; green horizontal bar indicates the 95% confidence interval (CI) for N1/K2(Q)L614A +N2B/K2(Q)L614A. Significant potentiation was observed when one of the two subunits included the L614A substitution and Q to R editing (P<0.0001, one-way ANOVA withpost hocStudent-Newman-Keuls comparison); 95% CI for N1/K2(Q)L614A +N2B/K2(R)L614A (yellow bar). Potentiation was greatest when both chimeric subunits were edited (R) and mutated (L614A); 95% C.I. for N1/K2(R)L614A+N2B/K2(R)L614A (pink bar). Figure 4: Intrasubunit interaction between the pore loop and M3 helix. Whole-cell current evoked by 10 μM NMDA and 10 μM glycine (open bars) at −80 mV before and after exposure to 30 μM DHA (solid bar) in cells co-transfected with N1/K2(R)+N2B/K2(Q)L614A ( a ), N1/K2(R)L614A+N2B/K2(Q)L614A ( b ), N1/K2(Q)+N2B/K2(R)L614A ( c ), or N1/K2(R)L614A+N2B/K2(R)L614A ( d ). ( e ) Plot of current evoked immediately after exposure to DHA as a fraction of control current before DHA (mean±s.e.m.) for the 12 chimeric constructs and, for comparison, homomeric L614A mutants of GluK2(Q) and (R). Sample size is shown for each bar. Note the logarithmic scale. DHA had minimal effect when L614A and Q to R editing were not present on the same chimeric subunit; green horizontal bar indicates the 95% confidence interval (CI) for N1/K2(Q)L614A +N2B/K2(Q)L614A. Significant potentiation was observed when one of the two subunits included the L614A substitution and Q to R editing ( P <0.0001, one-way ANOVA with post hoc Student-Newman-Keuls comparison); 95% CI for N1/K2(Q)L614A +N2B/K2(R)L614A (yellow bar). Potentiation was greatest when both chimeric subunits were edited (R) and mutated (L614A); 95% C.I. for N1/K2(R)L614A+N2B/K2(R)L614A (pink bar). Full size image Together, the results in Fig. 4 provide strong evidence that the Arg side chain in edited Q/R sites interacts with the residue at position 614 within the same subunit. Channels that included an edited (R) subunit wild type at L614 and an L614A mutation on the adjacent unedited (Q) subunit displayed no significant potentiation relative to completely unedited (Q/Q) combinations. However, combinations in which both subunits were edited (R) but only one of them bore the L614A mutation exhibited stronger potentiation than combinations with one or both subunits mutated (L614A) but only one subunit edited (R) ( P <0.0001, one-way ANOVA with post hoc Student-Newman-Keuls comparison) ( Fig. 4e ), suggesting that confinement of four Arg guanidinium groups within the pore enhances the interaction with M3. Thus, the effect of DHA is strongest when all four subunits are edited at the Q/R site, whether the effect is inhibition, as for wild-type L614, or potentiation, with either two or four L614A substitutions. Importantly, the Q/R site interaction with M3 is likely to be equivalent in both the A/C and B/D subunit pairs because a similar level of potentiation was observed for channels that included either the N1/K2(R)L614A or the N2B/K2(R)L614A constructs ( Fig. 5 ). The only evidence for asymmetry came from the N1/K2(R)L614A+N2B/K2(Q) combination that displayed weaker potentiation by DHA than any of the other constructs with L614A on an edited (R) subunit ( P =0.002, one-way ANOVA with post hoc Student-Newman-Keuls comparison) ( Fig. 4e ). Despite this difference, there was strong correlation between the effects of DHA on symmetric construct pairs ( Fig. 5b ) (Pearson correlation coefficient=0.925 for the 6 off-diagonal points; P =0.0083 that the association is invalid; regression line for the off-diagonal points in cyan and extended to the axes in red). Indeed, the relation between analogous pairs of N1/K2 and N2B/K2 constructs was well described by a model assuming fourfold radial symmetry ( F test) ( Fig. 5b , perfect symmetry indicated by the dashed line). 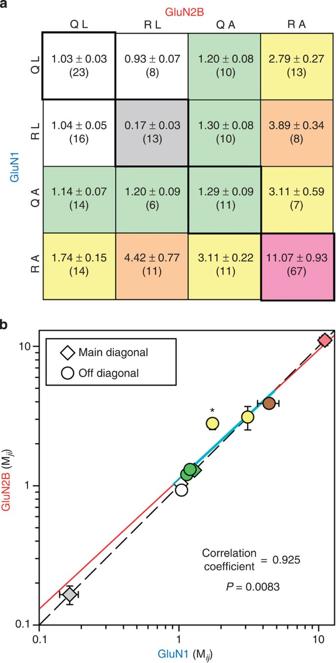Figure 5: Radial symmetry in chimeric receptor pores. (a) Interaction matrix for Q/R editing and L614A substitutions to chimeric N1/K2 and N2B/K2 subunits. Matrix elements displayIDHA/Icontrolas mean±s.e.m. (no. of cells). Colour code: No A+<2R, white; No A+2R, grey; A not with R, green; 1R with 1 or 2 A, yellow; 1A with 2R, tan; 2A with 2R, pink. (b) Diamonds plotIDHA/Icontrolfor the four main diagonal elements (Mjiversus Mijwherei=j) outlined in bold in (a). Circles plotIDHA/Icontrolin N2B/K2 versus N1/K2 for symmetric constructs (off-diagonal matrix elements, Mjiversus Mijand i≠j). Pearson product moment correlation coefficient=0.925 for the six off-diagonal points indicates strong symmetric association (P=0.0083 that the association is invalid). In addition, linear regression to the six off-diagonal matrix element points (solid line, 2 parameters) was not statistically superior (F test) to the line of identity through the symmetric main diagonal elements (dashed line, no free parameters). The solid line is shown in cyan over the range of off-diagonal points used for regression. It is extended to each axis in red. * only the N1/K2(Q) +N2B/K2(R)L614A, N1/K2(R)L614A+N2B/K2(Q) coordinate pair displayed significant asymmetry (P=0.002, one-way ANOVA withpost hocStudent-Newman-Keuls comparison). Figure 5: Radial symmetry in chimeric receptor pores. ( a ) Interaction matrix for Q/R editing and L614A substitutions to chimeric N1/K2 and N2B/K2 subunits. Matrix elements display I DHA / I control as mean±s.e.m. (no. of cells). Colour code: No A+<2R, white; No A+2R, grey; A not with R, green; 1R with 1 or 2 A, yellow; 1A with 2R, tan; 2A with 2R, pink. ( b ) Diamonds plot I DHA / I control for the four main diagonal elements (M ji versus M ij where i = j ) outlined in bold in ( a ). Circles plot I DHA / I control in N2B/K2 versus N1/K2 for symmetric constructs (off-diagonal matrix elements, M ji versus M ij and i≠j). Pearson product moment correlation coefficient=0.925 for the six off-diagonal points indicates strong symmetric association ( P =0.0083 that the association is invalid). In addition, linear regression to the six off-diagonal matrix element points (solid line, 2 parameters) was not statistically superior (F test) to the line of identity through the symmetric main diagonal elements (dashed line, no free parameters). The solid line is shown in cyan over the range of off-diagonal points used for regression. It is extended to each axis in red. * only the N1/K2(Q) +N2B/K2(R)L614A, N1/K2(R)L614A+N2B/K2(Q) coordinate pair displayed significant asymmetry ( P =0.002, one-way ANOVA with post hoc Student-Newman-Keuls comparison). Full size image Decoupling the co-agonist sites In addition to increasing agonist-evoked currents, in some cases exposure to DHA also increased the baseline holding current (for example, Figs 4d and 6a ). The magnitude of the change varied from cell to cell but on average was significantly larger for construct combinations that also showed the greatest potentiation of agonist-evoked current ( Fig. 6b ), raising the possibility that DHA was either increasing the open probability of unliganded chimeric channels [26] , [27] or enhancing channel activation by trace levels of agonist that might be present in our control external solution [20] , [21] , [28] . If the change in baseline involved activation by trace agonist levels, then it should be blocked or reversed by co-application of competitive antagonists, which was indeed the case for antagonists of the GluN1 glycine-binding site including ACEA 1021 (ref. 29 ) and 5-fluoro-indole-2-carboxylic acid (5F-I2CA) [30] , whereas competitive inhibitors of the GluN2 glutamate/NMDA-binding site, such as APV and CPP [31] , had less effect ( Fig. 6c,d ). 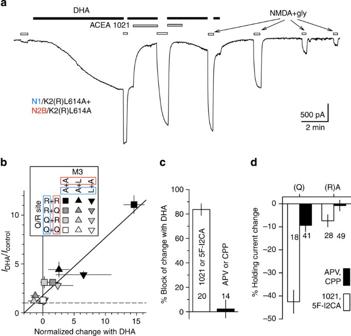Figure 6: Changes in holding current with DHA and antagonists. (a) Whole-cell current evoked by 10 μM NMDA and 10 μM glycine (open bars) before and after exposure to 15 μM DHA (black bars). The glycine site antagonist ACEA 1021 (1 μM) was applied together with DHA during the periods indicated by the grey bars. After the final exposure to DHA, the control external solution contained 0.1% BSA. (b) Plot of current evoked immediately after exposure to DHA (mean±s.e.m.) as a fraction of control current before DHA for the 12 chimeric constructs inFig. 4versus change in holding current with DHA exposure normalized to the current evoked by NMDA and glycine. Pearson product moment correlation coefficient=0.949 (P<0.0001). Sample size as given inFigs 4eand5a. (c) Percent block of DHA-induced change in holding current (mean±s.e.m.) for N1/K2(R)L614A+N2B/K2(R)L614A by 1 μM ACEA 1021 or 1 mM 5F-I2CA (20 cells) or by 50 μM APV or 30 μM CPP. Sample size is shown for each bar. (d) Percent change in baseline holding current (mean±s.e.m.) without DHA exposure. Figure 6: Changes in holding current with DHA and antagonists. ( a ) Whole-cell current evoked by 10 μM NMDA and 10 μM glycine (open bars) before and after exposure to 15 μM DHA (black bars). The glycine site antagonist ACEA 1021 (1 μM) was applied together with DHA during the periods indicated by the grey bars. After the final exposure to DHA, the control external solution contained 0.1% BSA. ( b ) Plot of current evoked immediately after exposure to DHA (mean±s.e.m.) as a fraction of control current before DHA for the 12 chimeric constructs in Fig. 4 versus change in holding current with DHA exposure normalized to the current evoked by NMDA and glycine. Pearson product moment correlation coefficient=0.949 ( P <0.0001). Sample size as given in Figs 4e and 5a . ( c ) Percent block of DHA-induced change in holding current (mean±s.e.m.) for N1/K2(R)L614A+N2B/K2(R)L614A by 1 μM ACEA 1021 or 1 mM 5F-I2CA (20 cells) or by 50 μM APV or 30 μM CPP. Sample size is shown for each bar. ( d ) Percent change in baseline holding current (mean±s.e.m.) without DHA exposure. Full size image Analysis of macroscopic [21] , [32] , [33] and single channel [34] , [35] , [36] currents suggest that efficient opening of wild-type NMDA receptor channels requires agonist occupancy of all four LBDs, with both GluN1 subunits binding glycine or D -serine and both GluN2 subunits binding glutamate or NMDA. In contrast, AMPA and kainate receptors can open with only a subset of the four agonist-binding sites occupied [37] , [38] , [39] . Our initial results with chimeric subunits showed that production of functional channels requires co-expression of N1/K2 and N2/K2 subunits ( Fig. 2a ) but did not determine whether simultaneous occupancy of both the glycine and NMDA sites is essential for channel activation. To test for channel activation by NMDA alone we recorded dose-response relations for NMDA in the presence of a glycine site antagonist (1 mM 5F-I2CA) and no added glycine and normalized to current evoked in the same cells by 1 mM NMDA plus 10 μM glycine and no antagonist ( Fig. 7a–d ). Currents were recorded both before and after exposure to DHA to see whether there was any change in apparent affinity or efficacy. 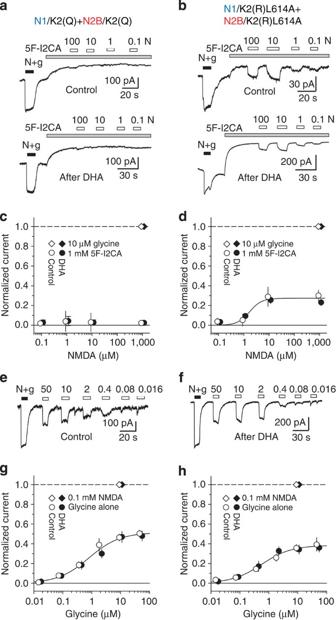Figure 7: Decoupling of co-agonist sites. (a,b) Whole-cell currents evoked by 1 mM NMDA and 10 μM glycine (solid bars), then by 1 mM, 10, 1 and 0.1 μM NMDA alone (open bars) in the presence of 1 mM 5F-I2CA, a glycine site antagonist (grey bars). N1/K2(Q)+N2B/K2(Q) (a) and N1/K2(R)L614A+N2B/K2(R)L614A (b) before (top) and after (bottom) exposure to 15 μM DHA. (c,d) Currents (mean±s.e.m.) evoked by NMDA alone plus 1 mM 5F-I2CA (circles) normalized to 1 mM NMDA plus 10 μM glycine (diamonds), before (open) and after (filled) exposure to DHA.Smooth curve:best Hill equation fit to NMDA alone (with 5F-I2CA) before and after DHA, EC50=1.7 μM,n=2.1 andImax=0.28 (6 cells). (e,f) Current evoked by 100 μM NMDA plus 10 μM glycine (solid bars), then by 50, 10, 2, 0.4, 0.08 and 0.016 μM glycine alone (open bars). Traces from N1/K2(Q)+N2B/K2(Q) before DHA (e) and from N1/K2(R)L614A+N2B/K2(R)L614A after DHA (f). (g,h) Currents (mean±s.e.m.) evoked by glycine alone (circles) normalized to 10 μM NMDA plus 10 μM glycine (diamonds), before (open) and after (filled) exposure to DHA.Smooth curves:best Hill equation fit to glycine alone before and after DHA for N1/K2(Q)+N2B/K2(Q) (g) with EC50=0.79 μM,n=0.82 andImax=0.51 (6 cells) and for N1/K2(R)L614A+N2B/K2(R)L614A (h) with EC50=0.57 μM,n=0.87 andImax=0.38 (10 cells). Exposure to DHA did not significantly alter the concentration response relations for NMDA alone (c,d) or glycine alone (g,h) (Ftest). For cells transfected with N1/K2(Q)+N2B/K2(Q), there was little evidence for channel activation by NMDA alone ( Fig 7a,c ; n =4 cells), either before or after DHA treatment. In contrast, NMDA alone evoked almost 30% as much current as NMDA plus glycine in cells co-transfected with the M3 mutant subunits N1/K2(R)L614A+ N2B/K2(R)L614A ( Fig. 7b,d ; n =6 cells). Moreover, treatment with DHA produced an equivalent increase in currents evoked by NMDA alone or with glycine, such that there was no significant change in the normalized dose-response relation ( Fig. 7d ; F test). Figure 7: Decoupling of co-agonist sites. ( a , b ) Whole-cell currents evoked by 1 mM NMDA and 10 μM glycine ( solid bars ), then by 1 mM, 10, 1 and 0.1 μM NMDA alone ( open bars ) in the presence of 1 mM 5F-I2CA, a glycine site antagonist ( grey bars ). N1/K2(Q)+N2B/K2(Q) ( a ) and N1/K2(R)L614A+N2B/K2(R)L614A ( b ) before ( top ) and after ( bottom ) exposure to 15 μM DHA. ( c , d ) Currents (mean±s.e.m.) evoked by NMDA alone plus 1 mM 5F-I2CA ( circles ) normalized to 1 mM NMDA plus 10 μM glycine ( diamonds ), before ( open ) and after ( filled ) exposure to DHA. Smooth curve: best Hill equation fit to NMDA alone (with 5F-I2CA) before and after DHA, EC 50 =1.7 μM, n =2.1 and I max =0.28 (6 cells). ( e , f ) Current evoked by 100 μM NMDA plus 10 μM glycine ( solid bars ), then by 50, 10, 2, 0.4, 0.08 and 0.016 μM glycine alone ( open bars ). Traces from N1/K2(Q)+N2B/K2(Q) before DHA ( e ) and from N1/K2(R)L614A+N2B/K2(R)L614A after DHA ( f ). ( g , h ) Currents (mean±s.e.m.) evoked by glycine alone ( circles ) normalized to 10 μM NMDA plus 10 μM glycine ( diamonds ), before ( open ) and after ( filled ) exposure to DHA. Smooth curves: best Hill equation fit to glycine alone before and after DHA for N1/K2(Q)+N2B/K2(Q) ( g ) with EC 50 =0.79 μM, n =0.82 and I max =0.51 (6 cells) and for N1/K2(R)L614A+N2B/K2(R)L614A ( h ) with EC 50 =0.57 μM, n =0.87 and I max =0.38 (10 cells). Exposure to DHA did not significantly alter the concentration response relations for NMDA alone ( c , d ) or glycine alone ( g , h ) ( F test). Full size image To test for channel activation by glycine alone, we recorded glycine dose-response relations in external solutions without added NMDA or glutamate ( Fig. 7e–h ), and in some cases including NMDA site competitive antagonists (either 50 μM APV or 30 μM CPP). Currents recorded before or after exposure to DHA were normalized to the control response evoked by 100 μM NMDA plus 10 μM glycine. In contrast to NMDA, application of glycine alone evoked substantial currents in cells expressing either the non-mutant N1/K2(Q)+N2B/K2(Q) (0.5 of control, n =6 cells) or the mutant N1/K2(R)L614A+N2B/K2(R)L614A chimeric subunits (0.4 of control, n =10 cells) ( Fig. 7e–h ). Importantly, there was little difference in the half-maximal dose (EC 50 ) for glycine between the two construct combinations (0.6 and 0.8 μM, respectively; t -test, P =0.52) and no significant change in the EC 50 following treatment with DHA ( F test). Collectively, these results suggest a loss of the strict requirement for all four agonist sites to be occupied in order for channels to open. Instead, chimeric channels that include the GluK2 TMD and linkers appear to be activated by glycine alone, or by NMDA alone for the M3 mutant constructs, with only a modest reduction in efficacy compared with co-application of both agonists together. The EC 50 values for activation of chimeric constructs by glycine or NMDA alone are somewhat lower than observed for intact wild-type subunits [29] or neuronal NMDA receptors [30] , [40] , which might reflect a difference in linkage from LBD to TMD [41] in the chimeric subunits, or alternatively, might be owing to the lack of negative allosteric coupling between agonist-binding sites [33] , [40] when only one agonist is applied. Our results support several conclusions about the structure and operation of iGluRs and their modulation by cis -unsaturated fatty acids. Despite minimal sequence identity [1] , the heteromeric extracellular ATD and LBD from NMDA receptor subunits GluN1 and GluN2B were able to operate the homomeric TMD from the GluK2 kainate receptor subunit, confirming the modular arrangement of iGluRs [42] , [43] , [44] . Moreover, the GluK2 TMD embedded within the chimeric subunits can completely reproduce the modulatory effects of DHA observed for full-length homomeric wild-type GluK2 (ref. 23 ) and for the M3 helix L614A point mutation in homomeric GluK2 channels [13] . These results strongly suggest that modulation of GluK2 by DHA involves a direct effect on the TMD via the membrane. In addition, our results provide strong evidence that an edited pore loop Q/R site Arg side chain interacts with the M3 helix [13] within an individual subunit rather than between adjacent subunits. Substantial potentiation by exposure to DHA was only observed when both Q to R editing and L614A substitution were present on the same chimeric subunit. Because a similar level of potentiation was observed for L614A substitution of either the N1/K2(R) or N2B/K2(R) subunits, our results also suggest that the pore retains fourfold radial symmetry in the open state, at least up to the level of the central cavity. Finally, our results demonstrate decoupling of the co-agonist sites in chimeric receptors, suggesting that linkage between the LBD and TMD underlies the strict requirement of intact wild-type NMDA receptors for occupation of both the agonist and co-agonist sites to promote channel opening (see also ref. 27 ). Previous work on chimeric iGluRs has involved transferring domains within the members of a subfamily (that is, GluN2A and GluN2B [45] , [46] or GluK1 and GluK2 (ref. 47 )) or between AMPA and kainate receptors [43] , [44] , which are more closely related to each other (~30–40% identity) than to any of the NMDA receptor subunits (<20% identity) [1] . Chimeric subunits with the M1-M3 segment from GluN1 transferred into GluK2 form functional homomeric channels [16] ; however, similar constructs using the M1-M3 portion of GluN2B are not functional as homomers and do not combine with the GluK2(GluN1 M1-M3) chimera [16] . Moreover, homomeric GluK2/GluN1 (M1-M3) channels do not exhibit voltage-dependent block by Mg [16] , which is a hallmark of native NMDA receptors [1] . On the basis of increasing evidence that the M4 transmembrane helix is essential for channel function [5] , [6] , [7] , we fused the entire TMD and extracellular linkers plus the cytoplasmic C-terminal tail of GluK2 to the extracellular ATD and LBD from GluN1 and GluN2B, including from the NMDA receptor subunits both the S1 segment preceding M1 and the extracellular S2 segment between M3 and M4 (ref. 42 ). Co-transfection of N1/K2+N2B/K2 subunits resulted in functional channels activated by NMDA and/or glycine. However, transfection of individual chimeric subunits alone failed to generate functional homomeric channels, consistent with the fact that NMDA receptors are obligate heteromers [1] and that the extracellular domains appear to play a major role in heteromer assembly [15] . Further experiments will be needed to determine whether chimeric subunits expressed alone fail to make it to the cell surface, or whether they assemble and transit to the surface as non-functional oligomers. Native iGluRs exhibit divergent modulation by AA and DHA. NMDA receptor-mediated currents potentiate two- to threefold by an increase in channel open probability [24] , [25] . Neuronal KA receptors [48] and fully edited recombinant channels [23] are strongly inhibited by AA and DHA, owing to a reduction in open probability [49] . Whereas AMPA receptors and recombinant KA receptors that include unedited (Q) wild-type subunits are relatively unaffected [23] , [50] . It remains unclear whether iGluR modulation by AA and DHA involves specific interaction with hydrophobic segments in the extracellular, intracellular or transmembrane portions of each subunit or whether it reflects sensitivity to changes in bulk properties of the membrane, analogous to the effect of membrane stretch on NMDA receptor gating [51] . Using chimeric constructs, wild type at M3 position L614, we found that the GluK2 TMD completely recapitulates the pattern of DHA modulation observed for full-length homo and heteromeric kainate receptors: strong inhibition of fully edited (R)/(R) channels, but little effect on channels that included unedited subunits. Significantly, there was no potentiation of unedited (Q)/(Q) chimeric channels, as might have been expected if DHA were to interact with hydrophobic regions of the NMDA receptor ATD, which are known to regulate activity of full-length NMDA receptors [15] , [52] . Although our results do not formally rule out such interactions with the ATD, they show that KA receptor modulation is completely determined by the TMD, suggesting that channel regulation likely depends on contacts within the membrane. Recent experiments on NMDA receptors [14] showed that unitary conductance, calcium permeability and the strength of magnesium block depend on an intersubunit interaction between a conserved M2 helix Trp residue in GluN1 and an M3 helix Ser (GluN2A and 2B) or Leu (GluN2C or 2D) in the adjacent GluN2 subunit (see Fig. 1d ). Work on homomeric kainate receptor channels formed by GluK2 has also provided evidence for interactions between the pore loop and residues along the M3 helix [13] ; however, our results in the present study indicate that interactions between Q/R site Arg residues and L614A at the level of the central cavity occur within an individual subunit rather than between adjacent subunits. In channels with one pair of edited (R) and one pair of unedited (Q) chimeric subunits, DHA caused strong potentiation only when the edited (R) subunits included the L614A mutation. Alanine substitution at L614 of unedited (Q) subunits had little or no effect regardless the mutation status at L614 of the adjacent edited (R) subunits. In contrast, channels with one pair of mutated (A) and one pair of wild type (L) subunits at position 614 exhibited stronger potentiation if both subunits were edited (R) than if the wild-type L614 subunits were unedited (Q), which may reflect interaction between adjacent Q/R site arginines in fully edited channels. By far the strongest potentiation occurred when an edited Q/R site and the L614A mutation were present on both chimeric subunit pairs, or on all four of the subunits in a homomeric full-length GluK2(R)L614A channel [13] . Agonist binding to iGluRs induces clam shell closure of the LBD [53] that is thought to open channels by exerting force on the extracellular ends of the transmembrane helices via short random coil linkers [3] . In the process of opening, portions of the TMD might convert from fourfold symmetry in the closed state to twofold symmetry in the open state [10] . A number of studies [8] , [27] , [41] provide evidence for asymmetries in and around the pore of NMDA receptors, but whether these reflect local effects of the substantial differences in primary sequence between GluN1 and GluN2 subunits ( Fig. 1d ) or more global dissimilarities in subunit conformation within the TMD remains uncertain [54] . Importantly, analysis of cadmium binding to homomeric GluA1 AMPA receptors with an Ala to Cys substitution in the conserved M3 SYTANL A AF motif (indicated by an open diamond in Fig. 1d ) provides evidence for twofold symmetry at the level of the bundle crossing [9] , which is thought to form the gate for ion flow. In the closed state crystal structure [3] , however, this conserved alanine lies right at the transition from twofold to fourfold symmetry. Thus, it remains to be determined whether the sharp closed state transition in symmetry is preserved in the open state or whether local twofold symmetry extends further down the transmembrane helices when channels open and/or desensitize [12] . The present study evaluates an interaction approximately three turns down the M3 helix in a zone of strong fourfold symmetry in the closed state [3] ; moreover, our results suggest that fourfold symmetry persists at this position when channels are open. This interpretation is most compatible with an alternating N1-N2-N1-N2 arrangement for chimeric subunits imposed by the extracellular NMDA receptor segments [15] . Although substantial evidence supports this organization [3] , [17] , [18] , there is also some data that instead favours an adjacent N1-N1-N2-N2 arrangement [5] , [19] , and our results cannot entirely exclude an adjacent organization. It is also notable that DHA regulates channels whether applied in the presence or absence of agonist, with kinetics of onset and recovery from modulation that are much slower than gating transitions [13] , [23] . Thus, it seems unlikely that our evidence for radial symmetry reflects a selective interaction that is exclusive to the fourfold symmetric closed state. Despite the fact that formation of functional channels requires co-expression of both chimeric N1/K2 and N2B/K2 subunits, our results show that currents can be activated by glycine alone, or in some cases NMDA alone, suggesting that the LBD does not dictate the strict requirement of intact NMDA receptors for dual occupancy by both agonists. Instead, it suggests that the need for all four agonist sites to be occupied depends on linkage between the LBD and TMD that is unique for NMDA receptors. Previous work on NMDA receptors with point mutations in GluN1 at the bundle crossing (replacement of alanine homologous to that in GluA1 mentioned above, see Fig. 1d ) also provided evidence for co-agonist site decoupling [27] , but mutations in this region are known to interfere with normal gating [26] . In contrast, L614, which was mutated to alanine in the present study, is well below the bundle crossing, and co-agonist site decoupling was also observed for the N1/K2(Q) +N2B/K2(Q) combination with no M3 mutations. Importantly, both KA and AMPA receptor channels can open with less than complete agonist occupancy [37] , [38] , [39] , and our results suggest that this property can be transferred by transplantation of the GluK2 TMD together with the short linkers that extend up to the LBD. Analysis of additional chimeric constructs with fusion joints closer to the TMD may reveal more about the structural basis for differential occupancy requirements between the iGluR family members. cDNA constructs and cell culture Subunit cDNAs, generously provided by Steve Heinemann, Peter Seeburg, Mark Mayer and Stefano Vicini, were all expressed from the pRK5 vector using the GluK2 signal sequence. Chimeric subunits were generated by a restriction enzyme (RE)-free PCR cloning method [55] or by ligation of PCR products with novel restriction sites inserted by silent mutations. The RE-free method involves two sense and two antisense primers for each joint that creates a 15 bp complementary overlap [55] (underlined). S1 to M1 joint: sense GluK2 CCCAATGGTACAAAC CCAGG and CCAGGCGTCTTCTCCTTCCTG, antisense GluN1 GTTTGTACCATTGGG CTTCTTGACCAAAATGGTCAGGC and CTTCTTGACCAAAATGGTCAGGC; antisense GluN2B GTTTGTACCATTGGG GCGAGATACCATGACACTGATGC and GCGAGATACCATGACACTGATGC. M3 to S2 joint: antisense GluK2 GTCAATGGGCGACTC CATGC and CATGCGTTCCACAGTCAGAAAGGC, sense GluN1 GAGTCGCCCATTGAC GGCATCAATGACCCCAGGCTC and GGCATCAATGACCCCAGGCTC, sense GluN2B GAGTCGCCCATTGAC GGCCTGAGTGACAAGAAGTTCC and GGCCTGAGTGACAAGAAGTTCC. S2 to M4 joint: sense GluK2 CCGGAGGAGGAGAGC AAAGAG and AAAGAGGCCAGTGCTCTGGG, antisense GluN1 GCTCTCCTCCTCCGG GCATTCCTGATACCGAACCC and GCATTCCTGATACCGAACCC, antisense GluN2B GCTCTCCTCCTCCGG GCAAATGCCAGTGAGCCAGAG and GCAAATGCCAGTGAGCCAGAG. M4 to CTD joint: sense GluN1 TGCC CAATTG AAGCAGATGCAGCTG and sense GluN2B GCAT CAATTG ATGGGTGTCTGTTCTGG primers generate Mfe I sites (bold) to match the endogenous unique site in GluK2. All constructs were sequenced by the Washington University PNACL facility. cDNAs were expressed by transient transfection in HEK 293 cells (ATCC) using lipofectamine 2000 (Invitrogen). The cells were propagated in 25 cm 2 flasks with MEM plus 10% fetal bovine serum and passaged once each week with protease XXIII (Sigma). Cells used for transfection were seeded onto 12-well plates and transfected the following day. Co-expression of GFP from a second vector was used to identify transfected cells. The day after transfection, cells were plated at low density on 35 mm plates that were coated with nitrocellulose; recordings were obtained on the following 2 days. Electrophysiology Cultures were bath perfused with Tyrode’s solution (in mM): 150 NaCl, 4 KCl, 2 MgCl 2 , 2 CaCl 2 , 10 glucose, 10 HEPES, pH 7.4 with NaOH. Whole-cell electrodes were pulled from borosilicate tubing (WPI) and filled with an internal solution that contained (in mM): 140 Cs-glucuronate, 10 EGTA, 5 CsCl, 5 MgCl 2 , 5 ATP, 1 GTP, 0.02 spermine and 10 HEPES, pH adjusted to 7.4 with CsOH. Agonists and antagonists were delivered in control extracellular solution (160 mM NaCl, 2 mM CaCl2 and 10 mM HEPES, pH adjusted to 7.4 with NaOH) by local perfusion from a multi-barrelled pipette positioned near the recorded cell. Currents were recorded with an Axopatch 200A amplifier controlled by p-Clamp software (Molecular Devices). Current-voltage relations were generated by averaging the currents recorded during a series of five ascending and descending membrane potential ramps (0.75 mV ms −1 ) [13] . Concentration response relations were fit with the Hill equation: I = I max /(1+(EC 50 /[agonist])^ n ). Results are presented as mean±s.e.m. and were considered significant for P <0.05. One-way ANOVA and t -tests were performed with SigmaStat (Systat Software). Curve fits using different numbers of parameters were evaluated by F -tests [13] . Molecular modelling Homology modelling of a receptor composed of two pair of chimeric subunits, N1/K2(R)+N2B/K2(R), was performed using modeller [56] release 9v7; available at http://salilab.org/modeller/ . The GluA2 tetramer crystal structure (PDB ID: 3KG2) was used as the template with sequence alignment from Fig. S2 of ref. 3 and twofold symmetry constraints for the A/C and B/D subunit pairs. How to cite this article: Wilding, T. J. et al. Radial symmetry in a chimeric glutamate receptor pore. Nat. Commun. 5:3349 doi: 10.1038/ncomms4349 (2014).